Mus81-Mms4 and Yen1 resolve a novel anaphase bridge formed by noncanonical Holliday junctions Downregulation of separase, condensin, Smc5/6, topoisomerase II and Cdc14 in Saccharomyces cerevisiae yields anaphase bridges formed by unresolved sister chromatids (SCBs). Here we report that the overlapping actions of the structure-selective endonucleases (SSEs) Mus81-Mms4/EME1 and Yen1/GEN1, but not Slx1-Slx4, are also essential to prevent the formation of spontaneous SCBs that depend on the homologous recombination pathway. We further show that the frequency of SCBs is boosted after mild replication stress and that they contain joint molecules enriched in non-canonical forms of the Holliday junction (HJ), including nicked-HJ (nHJ). We show that SCBs are mostly reversible upon activation of either Mus81-Mms4 or Yen1 in late anaphase, which is concomitant with the disappearance of non-canonical HJs and restoration of viable progeny. On the basis of these findings, we propose a model where unresolved recombination intermediates are a source of mitotic SCBs, and Mus81-Mms4 and Yen1 play a central role in their resolution in vivo . Failure to remove proteinaceous cohesion, topological catenations, or to complete DNA replication by mitosis in the budding yeast S. cerevisiae causes sister chromatid nondisjunction and the formation of anaphase bridges [1] , [2] , [3] , [4] , [5] . Importantly, anaphase bridges have been shown as a source of genetic instability linked to cancer onset and intratumour heterogeneity in humans [6] , [7] , [8] . Failure to timely process recombination intermediates in which sister chromatids are linked again through pairing of complementary strands, that is, forming joint molecules (JMs), is also expected to cause deleterious consequences in anaphase [8] , [9] . During the mitotic division, inter-sister recombination intermediates arise when the homologous recombination pathway (HR) is called on to repair several DNA insults such as double-strand breaks (DSBs), interstrand crosslinks, stalled replication forks (SRFs) and post-replicative gaps. In budding yeast, as well as in humans, the processing of JMs involves several helicases and at least three structure-selective endonucleases (SSEs): Slx1-Slx4, Mus81-Mms4 (EME1 in the fission yeast and humans) and Yen1 (GEN1 in humans) [9] , [10] , [11] . Among the helicases, the helicase–topoisomerase complex formed by the budding yeast helicase Sgs1 (Bloom’s syndrome BLM in humans), the type I topoisomerase Top3 (TOPOIIIα) and the cofactor Rmi1 (RMI1-RMI2) is by far the most studied in JM resolution [9] , [10] , [11] , [12] . This complex (hereafter refer to as STR) appears active throughout the cell cycle and removes JMs mainly through a process known as double Holliday junction (dHJ) dissolution [12] . The dHJ is the archetypical JM that arises when HR repairs a two-ended DSB by the so-called DSB repair pathway [13] , [14] , [15] . HR can also lead to other types of JMs as a consequence of DSBs being one-ended, DSBs being repaired by other pathways, or HR being called on to bypass SRFs, fill post-replicative gaps and so on [9] , [13] , [16] . In many of these cases, dHJs are not generated but, instead, other JMs, such as D-loops, and single intact or nicked Holliday junctions (iHJ and nHJ, respectively) are the intermediates that physically link the sister chromatids [9] , [10] , [11] , [13] , [16] . Several lines of evidence support that single iHJ and nHJ are mainly processed by SSEs, and that SSEs also backup STR in the processing of dHJs and other helicases in the processing of D-loops [9] , [10] , [11] , [16] . Thus, null mutants for SLX4 , MMS4 and MUS81 are synthetically lethal with the genes that encode the STR complex [17] . Besides, double-mutant combinations for different SSEs, or the SSEs and the STR, greatly increase the in vivo steady–state levels of JMs, not only in yeast but also in humans and flies [18] , [19] , [20] , [21] , [22] , [23] , [24] , [25] . Last, several in vitro studies have shown that SSEs can efficiently process prototypical JMs such as D-loops, iHJs and nHJs. For instance, Mus81-Mms4(EME1) from S. cerevisiae , and also from other eukaryotes, efficiently processes D-loops and nHJs [25] , [26] , [27] ; Yen1/GEN1 is thought to be the analogous of prokaryotic RuvC HJ resolvase and mainly processes iHJs [28] , whereas Slx1-Slx4 is a more promiscuous SSE whose function appears more related to overcome problems arising during DNA replication [18] , [29] . In addition, in vivo studies have also placed the regulatory subunit Slx4 as a component of other Slx1-independent SSE activities. Thus, very recently, mammalian SLX4 has been suggested to regulate the activity and specificity of the MUS81-EME1 and XPF-ERCC1 (refs 30 , 31 , 32 , 33 ), whereas yeast Slx4 appears to associate with the Rad1-Rad10 flap endonuclease [34] . In this work, we aim to determine whether persistent JMs, more specifically those that depend on SSEs for their resolution, cause anaphase bridges in anaphase. To this purpose, we modify the steady–state levels of these JMs by deleting different combinations of the yeast SSE genes together with exogenously forcing the cells to bypass replication stress by calling on HR. We find that both Mus81-Mms4 and Yen1, but not Slx4-related SSEs, are essential and compensate each other in preventing and resolving a new type of sister chromatid anaphase bridge, which mostly comprises noncanonical (discontinuous) forms of the HJ molecule. Mus81-Mms4 and Yen1 co-work to prevent missegregation With the objective of determining whether persistent JMs were a source of anaphase bridges, we began this work by testing whether an increase in the SRF and JM steady-state levels caused anaphase problems in Saccharomyces cerevisiae. As a reference, we used a cdc15-2 strain in which the chromosome XII right arm (cXIIr) telomere was labelled with a green fluorescent dot [5] , [35] , [36] . We reasoned that this strain would allow us to microscopically visualize a plethora of aberrant anaphase phenotypes that might arise once we modify the basal levels of SRFs and JMs. First, the cdc15-2 temperature-sensitive allele blocks the cell cycle in telophase when the temperature is shifted to 37 °C. As mother and daughter cells remain together at the block, the segregation outcome of all mitoses can be easily followed. Of note, this block also helps in stabilizing any anaphase bridge present as cytokinesis is also prevented [36] . Second, cXIIr is the longest and most segregation-challenging chromosome arm in the yeast genome as it carries the highly transcribed ribosomal DNA locus (rDNA) [5] , [35] , [36] , [37] . Accordingly, it forms the most frequent single segregation defect in yeast, often invisible by DAPI staining, although clearly evident when labelling distal regions in the arm [4] , [5] , [35] , [36] , [37] , [38] , [39] , [40] . Aside from being rich in catenations, the rDNA is a natural place for SRFs and a hot-spot for spontaneous JMs [41] , [42] , [43] . Hence, we hypothesized that if persistent SRFs and/or JMs posed a problem for sister chromatid segregation, cXIIr would be the best single chromosome arm to look at. To increase the SRF and JM steady–state levels we used the alkylating agent MMS and made single, double and triple mutants for the three SSEs expected to resolve JMs in eukaryotes [9] , [10] , [11] , [44] . We first observed that the cell cycle profile in response to MMS was not very different between the reference cdc15-2 strain and the SSE mutant combinations ( Supplementary Figs 1–3 and left-most panel in Fig. 1a ). Thus, in a dose–response experiment carried out on a synchronous G1-to-telophase cell cycle ( Supplementary Fig. 1 ), MMS concentrations higher than 0.03% (v/v) caused cells to stay in G1 in all cases, whereas most cells got arrested in G2/M at 0.01%, and only concentrations below this value (that is, 0.004% or lower) allowed cells to enter anaphase. In addition, a G1-to-telophase time-course showed that the S-phase window (from minutes 30 to 90) and the anaphase onset (at ~90 min) were equivalent for the reference and all SSE mutant strains in the absence of MMS ( Supplementary Figs 2 and 3 ). The presence of 0.004% MMS did not basically change the timing of these cell cycle events. Only in the slx4 Δ combinations there was a slight delay (~15–30 min) and a minor decrease in cells able to reach anaphase (~25%), which were not enhanced when the other SSEs were also deleted ( Supplementary Figs 2 and 3 , and Fig. 1a ). This behaviour in the slx4 Δ-carrying strains is likely due to the additional Slx4 role as an anti-checkpoint protein [45] . The overall conclusion from the cell cycle profiles is that at least the mms4 Δ and yen1 Δ mutant combinations do not abolish the G1/S and G2/M DNA damage checkpoints triggered on MMS treatment, nor do they lead to their hyperactivation. 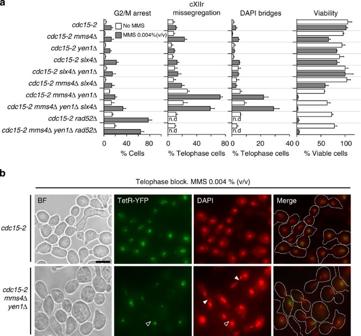Figure 1: Combined deletion ofMMS4andYEN1causes Rad52-dependent spontaneous and MMS-induced anaphase bridges. Overnight cultures of the strain FM588 (cdc15-2 Tel-cXIIr:tetO tetR-YFP), knocked out single-mutant derivatives of FM588 forRAD52,SLX4,MMS4andYEN1, double mutants combinations for the endonucleases and the triple mutantsslx4Δmms4Δyen1Δ andmms4Δyen1Δrad52Δ were first arrested in G1 at 25 °C. They were then split into two media, one of them containing MMS 0.004% (v/v), and finally released into a synchronous cell cycle at 37 °C for 4 h. (a) Percentage of cells that did not pass G2/M (left-most panel), chromosome XII missegregation (left-middle panel), DAPI-stained anaphase bridges (right-middle panel) and viable progeny after the telophase release (right-most panel) (mean±s.e.m.,N=3). DAPI-stained anaphase bridges and chromosome XII (cXII) missegregation are relative to cells able to reach telophase, that is, cells that passed G2/M. Open bars plot results obtained without exogenously induced DNA damage, whereas filled bars plot results upon 0.004% (v/v) MMS treatment. Strains carryingrad52Δ did not pass G2/M in MMS and therefore cXII missegregation and DAPI-stained bridges could not be determined (n.d.). (b) Representative micrographs of z-stack maximum projections from the telophase block of thecdc15-2and thecdc15-2 mms4Δyen1Δ strains in MMS 0.004% (v/v). White full triangles point to DAPI-stained anaphase bridges and white open triangles point to DAPI-invisible anaphase bridges comprising cXIIr (see text for details andFig. 3for further support). Scale bar in bright field (BF) micrograph represents 5 μm. Figure 1: Combined deletion of MMS4 and YEN1 causes Rad52-dependent spontaneous and MMS-induced anaphase bridges. Overnight cultures of the strain FM588 ( cdc15-2 Tel-cXIIr:tetO tetR-YFP ), knocked out single-mutant derivatives of FM588 for RAD52 , SLX4 , MMS4 and YEN1 , double mutants combinations for the endonucleases and the triple mutants slx4 Δ mms4 Δ yen1 Δ and mms4 Δ yen1 Δ rad52 Δ were first arrested in G1 at 25 °C. They were then split into two media, one of them containing MMS 0.004% (v/v), and finally released into a synchronous cell cycle at 37 °C for 4 h. ( a ) Percentage of cells that did not pass G2/M (left-most panel), chromosome XII missegregation (left-middle panel), DAPI-stained anaphase bridges (right-middle panel) and viable progeny after the telophase release (right-most panel) (mean±s.e.m., N =3). DAPI-stained anaphase bridges and chromosome XII (cXII) missegregation are relative to cells able to reach telophase, that is, cells that passed G2/M. Open bars plot results obtained without exogenously induced DNA damage, whereas filled bars plot results upon 0.004% (v/v) MMS treatment. Strains carrying rad52 Δ did not pass G2/M in MMS and therefore cXII missegregation and DAPI-stained bridges could not be determined (n.d.). ( b ) Representative micrographs of z-stack maximum projections from the telophase block of the cdc15-2 and the cdc15-2 mms4 Δ yen1 Δ strains in MMS 0.004% (v/v). White full triangles point to DAPI-stained anaphase bridges and white open triangles point to DAPI-invisible anaphase bridges comprising cXIIr (see text for details and Fig. 3 for further support). Scale bar in bright field (BF) micrograph represents 5 μm. Full size image Remarkably, we did observe frequent anaphase abnormalities for several SSE mutants, especially when they were treated with MMS ( Fig. 1a , two central panels, and Fig. 1b ). These anaphase problems were mostly observed in the form of cXIIr missegregation and less frequently as DAPI-stained bridges. Thus, the mms4 Δ mutant missegregated cXIIr in up to 20% of the anaphases on low MMS exposure, and this situation was exacerbated in the double mutant mms4 Δ yen1 Δ. In this mutant, cXIIr missegregation was around 25% in the absence of MMS and 70% in its presence. In addition, 30% of the cells with missegregated cXIIr in MMS also contained DAPI-stained bridges ( Fig. 1b ). Interestingly, the missegregation of cXIIr appeared as an end point outcome in all cases; that is, no transient higher peaks of missegregation were seen throughout the time-course ( Supplementary Fig. 3 ). In agreement with these anaphase abnormalities, the viability of the progeny after a telophase release (right-most panel in Fig. 1a ) or on continuous growth in 0.004% MMS ( Supplementary Fig. 4a ) was greatly reduced in the mms4 Δ yen1 Δ combinations. Interestingly, the progeny for the mms4 Δ yen1 Δ double mutant developed into microcolonies ranging from four to more than fifty cells before becoming unviable in MMS ( Supplementary Fig. 4b ). Strikingly, deletion of SLX4 did not enhance the observed anaphase abnormalities in any case. This latter result differs from very recent findings in humans showing that SLX4 and GEN1 play the major role in preventing DAPI-stained anaphase bridges [30] , [31] . Noteworthy, human SLX4 interacts with MUS81-EME1 (refs 30 , 31 , 32 ), a feature not reported at first in yeast [46] . Although we reasoned that by deleting SLX4 we were covering all known yeast Slx4-related SSE activities (that is, Slx1-Slx4 and Rad1-Rad10-Slx4) [34] , the cell cycle delay of the slx4 Δ combinations prompted us to further use slx1 Δ to confirm that the Slx1-Slx4 complex had no role in preventing the missegregation of cXIIr and the DAPI-stained bridges. Indeed, the different slx1 Δ combinations did not differ from their SLX1 counterparts ( Supplementary Fig. 5 ). Altogether, we concluded from these experiments that Mus81-Mms4 and Yen1, but not Slx1-Slx4, jointly contribute to the faithful segregation of chromosomes in anaphase. Correspondingly, we also propose that loss of viability in mms4 Δ yen1 Δ mutants likely occurs through mitotic catastrophe (see also below) and that previous observations of a G2/M arrest in the double mutant after prolonged MMS exposure likely accounts for DNA damage sensed in daughter cells that have suffered from such catastrophe [36] , [47] . Besides, our cytological results point out that at least part of the genetic instability previously associated with the mus81 Δ yen1 Δ double mutant may be caused after passing through aberrant mitoses rather than mistakenly resolving JMs, also in agreement with previous observations [21] . The mms4 Δ yen1 Δ mutant carries anaphase-persistent JMs We next addressed whether the anaphase problems observed in the mms4 Δ yen1 Δ double mutant were due to the presence of persistent SRFs or JMs. To discern between SRFs and JMs, we looked at whether the anaphase problems genetically depended on HR. As HR is called on to bypass SRFs at the expense of producing JMs behind the restored RFs, HR-defective strains are expected to increase their SRF steady–state levels (or DSBs after SRF collapse) and decrease the JM levels [43] . We thus deleted RAD52 , a central gene in HR, in the mms4 Δ yen1 Δ combinations. This deletion happened to yield a G2/M arrest and a substantial loss of viability in the presence of even very low MMS concentrations ( Supplementary Figs 1–3 and Fig. 1 ). Hence, we only determined whether rad52 Δ mms4 Δ yen1 Δ rescued the cXIIr missegregation phenotype of mms4 Δ yen1 Δ in an MMS-free media, which was the case ( Fig. 1a , lowest two bars). We concluded that an increase of spontaneous JMs in mms4 Δ yen1 Δ, and not persistent SRFs, was the cause of the observed 25% cXIIr missegregation (see below for further support). Next, we employed pulse-field gel electrophoresis (PFGE) to achieve several goals based on the fact that branched DNA structures preclude chromosomes from running in a PFGE [21] , [48] . This approach has been used before to show that the mus81 Δ yen1 Δ double mutant bears persistent MMS-dependent JMs in G2-blocked cells [21] . First, we wondered whether chromosome XII (cXII), and other chromosomes, still had JMs in anaphase, or rather, cXIIr missegregation was an indirect consequence of a transient increase in JMs during S/G2. Second, we intended to determine which chromosomes were more prone to have persistent JMs. Last, we wanted to check whether cXII broke down when cells entered anaphase. Thus, we observed that the intensity of cXII able to enter the gel greatly faded away for the mms4 Δ yen1 Δ strain in MMS ( Fig. 2a ). Relative intensity among chromosomes also showed that cXII was more severely affected than any other and that cIV, the second largest chromosome, was somewhat affected as well ( Fig. 2b ). Finally, we could not see evidence of chromosome breakage for cXII using a probe against the rDNA, rather cXII remained trapped in the well in the mms4 Δ yen1 Δ strain upon MMS treatment ( Fig. 2a ). As mentioned above, entrapment within the well is indicative of branched DNA structures. 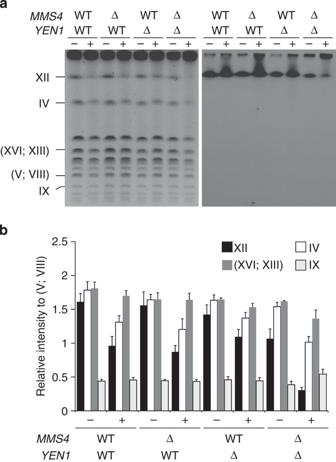Figure 2: Mms4 and Yen1 compensate one another in resolving chromosomes XII and IV sister chromatids DNA-DNA linkages on ongoing DNA damage. Strains FM588 (cdc15-2 Tel-cXIIr:tetO tetR-YFP) and its derivatives carrying eithermms4Δ oryen1Δ, plus the double mutantmms4Δyen1Δ, were treated as inFig. 1. (a) Pulsed-field gel electrophoresis (PFGE) of all yeast chromosomes at thecdc15-2telophase block. Left picture: gel after ethidium bromide staining. Right picture: Southern blot of that gel against an rDNA probe, that is, cXII. (b) Quantitation of chromosome bands for XII, IV, XVI+XIII and IX relative to the V+VIII chromosome band intensity. The plot is from the gel shown plus two more independent experiments (mean±s.e.m.,N=3). The minus and plus signs represent the absence of MMS or the presence of 0.004% (v/v) MMS in the cultures, respectively. Figure 2: Mms4 and Yen1 compensate one another in resolving chromosomes XII and IV sister chromatids DNA-DNA linkages on ongoing DNA damage. Strains FM588 ( cdc15-2 Tel-cXIIr:tetO tetR-YFP ) and its derivatives carrying either mms4 Δ or yen1 Δ, plus the double mutant mms4 Δ yen1 Δ, were treated as in Fig. 1 . ( a ) Pulsed-field gel electrophoresis (PFGE) of all yeast chromosomes at the cdc15-2 telophase block. Left picture: gel after ethidium bromide staining. Right picture: Southern blot of that gel against an rDNA probe, that is, cXII. ( b ) Quantitation of chromosome bands for XII, IV, XVI+XIII and IX relative to the V+VIII chromosome band intensity. The plot is from the gel shown plus two more independent experiments (mean±s.e.m., N =3). The minus and plus signs represent the absence of MMS or the presence of 0.004% (v/v) MMS in the cultures, respectively. Full size image Re-activation of either Mms4 or Yen1 resolves JMs and SCBs Next, we addressed whether the cXIIr missegregation phenotype was reversible on addition of either SSE in telophase-blocked cells ( Fig. 3 ). This is an important issue as the actual cause of the observed cXIIr missegregation could be due to either cXIIr breakage or unresolved cXIIr sister chromatids. The fact that we did not see a fragmented cXII in a PFGE supports the latter. Nevertheless, it was puzzling that we did not see transient cXIIr missegregation in the time-courses ( Supplementary Fig. 3 ), nor did we observe DAPI-stained bridges for a significant proportion of anaphases with missegregated cXIIr ( Fig. 1 ). It is worth mentioning though that an anaphase bridge formed by just the cXIIr is poorly stained by DAPI [36] . Furthermore, a novel type of DAPI-invisible anaphase bridge has been described in higher eukaryotes [8] , [49] . It may well happen that cXIIr was forming one of these DAPI-invisible anaphase bridges. We reasoned that if cXIIr sister chromatids were part of an anaphase bridge, there was a chance of reversing cXIIr missegregation on JM resolution, as we have shown previously in the case of topological entanglements [35] , [36] . On the contrary, a broken cXIIr would make missegregation necessarily irreversible. Thus, we carried out the G1-to-telophase experiment with and without MMS in two strains that respectively bore mms4 Δ GAL-YEN1 and GAL-MMS4 yen1 Δ. In raffinose both strains are like the mms4 Δ yen1 Δ double mutant because they do not express the corresponding gene under the GAL promoter. Once they reached telophase, galactose was added to express the GAL-controlled gene. Strikingly, the cXIIr missegregation phenotype was reverted in both strains, as was the presence of DAPI-stained bridges in MMS ( Fig. 3a ). This was not the case in the mms4 Δ yen1 Δ strain, ruling out any side effect due to the sugar switch. Noteworthy, the resolution and segregation of cXIIr correlated with the ability of cXII to re-enter a PFGE ( Fig. 3b,c ) and to a better offspring viability ( Fig. 3d ). From this experiment we concluded that the observed cXIIr missegregation is due to an anaphase bridge formed by the sister chromatids of that chromosome arm that remain partly unresolved in telophase, that is, cXIIr forms a sister chromatid anaphase bridge (SCB) in the mms4 Δ yen1 Δ strain. Importantly, we also got further support for this bridge being formed by JMs instead of SRFs as cleavage of the latter by either SSE would break cXIIr while pulling sisters apart, and thereby no cXIIr-Tel segregation, no intact cXII in PFGE and no viable progeny would be obtained. Correspondingly, continuous overexpression of either MMS4 or YEN1 was not toxic; rather, it conferred resistance to MMS ( Supplementary Fig. 6 ), a result that does not fit well with Mus81-Mms4 or Yen1 being deregulated to cut RFs when overproduced. 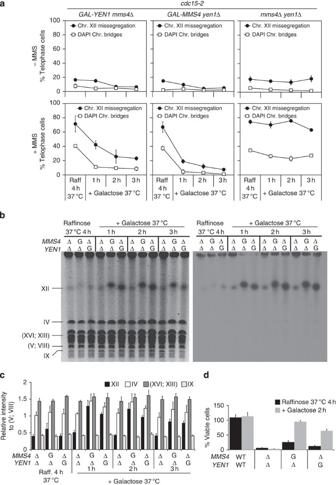Figure 3: DAPI-stained anaphase bridges, missegregation of chromosome XII and DNA-DNA linkages observed in the double mutantmms4Δyen1Δ are all reverted upon overexpression of either of the two resolvases at the telophase block. Strains FM1185 (cdc15-2 Tel-cXIIr:tetO tetR-YFP mms4Δyen1Δ), FM1428 (cdc15-2 Tel-cXIIr:tetO tetR-YFP GAL-MMS4 yen1Δ) and FM1432 (cdc15-2 Tel-cXIIr:tetO tetR-YFP mms4ΔGAL-YEN1) were treated as inFig. 1except for the sugar source, which was raffinose instead of glucose. At the telophase block, galactose was added to induce the respective GAL-driven endonuclease gene and samples were taken at the indicated time points. (a) Time course of the segregation status of cXIIr and the disappearance of DAPI-stained bridges after galactose addition (mean±s.e.m.,N=3). (b) Pulsed-field gel electrophoresis for large yeast chromosomes during the GAL induction time course in the presence of 0.004% (v/v) MMS. Left picture: gel after ethidium bromide staining. Right picture: Southern blot of that gel against an rDNA probe. (c) Quantitation of chromosome bands for XII, IV, XVI+XIII and IX relative to the V+VIII band intensity. The plot is from the gel shown in (b) plus two more independent experiments (mean±s.e.m.,N=3). (d) Viability of cells released from telophase before and 2 h after the galactose addition (mean±s.e.m.,N=3). The delta symbol denotes a knockout for the referred gene and the letter G indicates that the gene is under theGAL1promoter. Figure 3: DAPI-stained anaphase bridges, missegregation of chromosome XII and DNA-DNA linkages observed in the double mutant mms4 Δ yen1 Δ are all reverted upon overexpression of either of the two resolvases at the telophase block. Strains FM1185 ( cdc15-2 Tel-cXIIr:tetO tetR-YFP mms4 Δ yen1 Δ), FM1428 ( cdc15-2 Tel-cXIIr:tetO tetR-YFP GAL-MMS4 yen1 Δ) and FM1432 ( cdc15-2 Tel-cXIIr:tetO tetR-YFP mms4 Δ GAL-YEN1 ) were treated as in Fig. 1 except for the sugar source, which was raffinose instead of glucose. At the telophase block, galactose was added to induce the respective GAL-driven endonuclease gene and samples were taken at the indicated time points. ( a ) Time course of the segregation status of cXIIr and the disappearance of DAPI-stained bridges after galactose addition (mean±s.e.m., N =3). ( b ) Pulsed-field gel electrophoresis for large yeast chromosomes during the GAL induction time course in the presence of 0.004% (v/v) MMS. Left picture: gel after ethidium bromide staining. Right picture: Southern blot of that gel against an rDNA probe. ( c ) Quantitation of chromosome bands for XII, IV, XVI+XIII and IX relative to the V+VIII band intensity. The plot is from the gel shown in ( b ) plus two more independent experiments (mean±s.e.m., N =3). ( d ) Viability of cells released from telophase before and 2 h after the galactose addition (mean±s.e.m., N =3). The delta symbol denotes a knockout for the referred gene and the letter G indicates that the gene is under the GAL1 promoter. Full size image JMs at the rDNA in mms4 Δ yen1 Δ comprise non-canonical HJs A key mechanistic insight into how JMs might get resolved by these SSEs could also be derived from the above experiment. As Mus81-Mms4 and Yen1 can largely suppress the aberrant phenotypes of the double mutant in late anaphase, they must process similar or dynamically interchangeable anaphase-stable JMs. This is a critical issue as many reports have highlighted that Mus81-Mms4/EME1 and Yen1/GEN1 process different JMs in vitro [26] , [27] , [28] , [46] , [50] , [51] . Hence, we now focused our efforts on the physical nature of JMs in the mms4 Δ yen1 Δ telophase block and after induction of either SSE. To this aim, we studied the branched DNA structures present within the rDNA sequence. As mentioned, we expected the rDNA to be the most important JM hot-spot [42] , [43] , and so suggest the microscopy and PFGE results ( Figs 1 and 2 ). Neutral, neutral two-dimensional DNA electrophoresis (NN-2D) is the reference technique to assess the physical nature of branched DNA structures. NN-2D has been recently used to show that the mus81 Δ yen1 Δ double mutant bears higher levels of DSB-dependent X-shaped JMs in G2-blocked cells [23] , [25] . When we performed NN-2D for all telophase blocks, we observed a clear correlation between the severity of cXIIr missegregation and the spike that corresponds to X-shaped molecules ( Fig. 4a,b ). Noteworthy, the spike disappeared almost completely upon induction of either MMS4 or YEN1 in telophase ( Fig. 4c,d ). 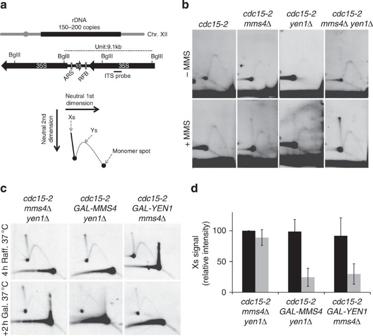Figure 4: X-shaped molecules are the main source of the DNA-DNA linkages observed in telophase-blocked cells deficient for both Mus81-Mms4 and Yen1. (a) A schematic of the chromosome XII rDNA array and the BglII rDNA fragment chosen for the NN-2Ds. The branched DNA molecules detectable with a probe against the selected BglII fragment is depicted underneath (Xs, HJs, hemicatenanes and so on; Ys, replication forks, single-end invasions and so on). (b) The strain FM588 (cdc15-2 Tel-cXIIr:tetO tetR-YFP) and its derivatives carrying eithermms4Δ oryen1Δ, plus the double mutantmms4Δyen1Δ, were treated as inFig. 1. Samples taken at the telophase block were processed for NN-2D to assess the physical nature of the branched DNA molecules. (c) The strain FM1185 (cdc15-2 Tel-cXIIr:tetO tetR-YFP mms4Δyen1Δ) and derivatives carrying eitherGAL-MMS4 yen1Δ ormms4ΔGAL-YEN1were treated as inFig. 3. Samples taken at the telophase block in raffinose and 2 h after galactose addition were processed for NN-2D as in (b). (d) Quantitation of the normalized amounts of the X-shaped molecules relative to themms4Δyen1Δ strain before the GAL induction (mean±s.e.m.,N=3). Dark and light grey bars depict relative signals before and after the GAL induction, respectively. Figure 4: X-shaped molecules are the main source of the DNA-DNA linkages observed in telophase-blocked cells deficient for both Mus81-Mms4 and Yen1. ( a ) A schematic of the chromosome XII rDNA array and the BglII rDNA fragment chosen for the NN-2Ds. The branched DNA molecules detectable with a probe against the selected BglII fragment is depicted underneath (Xs, HJs, hemicatenanes and so on; Ys, replication forks, single-end invasions and so on). ( b ) The strain FM588 ( cdc15-2 Tel-cXIIr:tetO tetR-YFP ) and its derivatives carrying either mms4 Δ or yen1 Δ, plus the double mutant mms4 Δ yen1 Δ, were treated as in Fig. 1 . Samples taken at the telophase block were processed for NN-2D to assess the physical nature of the branched DNA molecules. ( c ) The strain FM1185 ( cdc15-2 Tel-cXIIr:tetO tetR-YFP mms4 Δ yen1 Δ) and derivatives carrying either GAL-MMS4 yen1 Δ or mms4 Δ GAL-YEN1 were treated as in Fig. 3 . Samples taken at the telophase block in raffinose and 2 h after galactose addition were processed for NN-2D as in ( b ). ( d ) Quantitation of the normalized amounts of the X-shaped molecules relative to the mms4 Δ yen1 Δ strain before the GAL induction (mean±s.e.m., N =3). Dark and light grey bars depict relative signals before and after the GAL induction, respectively. Full size image As mentioned before, a key difference between Mus81-Mms4 and Yen1 is the in vitro preference they show for the HJ substrate [27] , [28] , [46] . Thus, Mus81-Mms4 preferentially cleaves a HJ with a nick very close to the junction (nHJ), whereas Yen1 cleaves the intact HJ (iHJ). Having shown that either SSE resolves most of the X-shaped spike in vivo , we wondered whether they were both acting on the same substrates and whether iHJs and nHJs actually coexisted in the 2D spike. To address this, we run a third alkaline dimension to our NN-2Ds (NNA-3D) [52] . DNA denaturation would cause an iHJ to split into four identical single-stranded DNA molecules (ssDNA), whereas nHJs would split into three identical ssDNAs plus one (symmetrical nHJ) or two (asymmetrical nHJ) smaller ssDNAs ( Supplementary Fig. 7 for a schematic). Strikingly, we observed in the mms4 Δ yen1 Δ X-shaped spike the NNA-3D pattern expected for nHJs with the nick located just at the junction ( Fig. 5a,b and Supplementary Fig. 7 ). When we measured the normalized intensities between the full-length ssDNAs and the sum of the smaller ssDNAs, we obtained a ratio of 2.86±0.17 (mean±s.e.m., N =11). This value is strikingly very close to the 3:1 ratio expected if all X-shaped molecules were nHJs ( Supplementary Fig. 7 ). To shed more light on this structure we further subjected the samples to the action of the purified bacterial HJ resolvase RuvC and the T4 DNA ligase ( Fig. 5c ). With these assays we intended to address two issues: first, to corroborate that the X-shaped spike was actually a HJ and not a hemicatenane and, second, to biochemically test whether the discontinuity in one of the strands was actually a nick or, rather, it may correspond to a small gap (impossible to differentiate from the NNA-3D profile). Hemicatenanes, which are recombination intermediate that might also link two sister chromatids, comigrate with HJs in the NN-2D spike and are expected to comigrate with the full-length ssDNAs in the NNA-3D. Although the 3:1 ratio in the NNA-3D strongly suggests the absence of hemicatenanes, as well as iHJs, we decided to treat our samples with RuvC, which has been traditionally used to distinguish between HJs and hemicatenanes [43] , [53] . Importantly, RuvC cuts both iHJs and nHJs [54] . Hence, we wondered whether any of the X-shaped molecules observed in the mms4 Δ yen1 Δ mutant were resistant to RuvC, but found that all X-shaped DNA disappeared on RuvC treatment ( Fig. 5c ), supporting the idea that the observed X-shaped molecules are HJs. To distinguish between nHJs and any HJ whose discontinuous strand actually carries a small gap, we tested whether previous treatment with T4 DNA ligase abolished the splitting of the X-shaped spike in the NNA-3D. Although we could not achieve complete absence of the smaller ssDNAs in the NNA-3D ( Fig. 5c ), the full/partial-length ssDNA ratio rose to 7:1, suggesting that at least half of the discontinuous HJs are ligatable nHJs. The other half might be unligatable nHJs, HJs with small gaps and/or due to an incomplete reaction of the ligase. Finally, we wondered whether these X-shaped JMs were resolved on expression of either SSE in telophase, and thus correlated with the previous observation of unlinkage and segregation of cXII ( Fig. 3 ). Indeed, we found that these JMs largely disappeared on induction of either GAL-MMS4 or GAL-YEN1 in telophase ( Fig. 5d ). 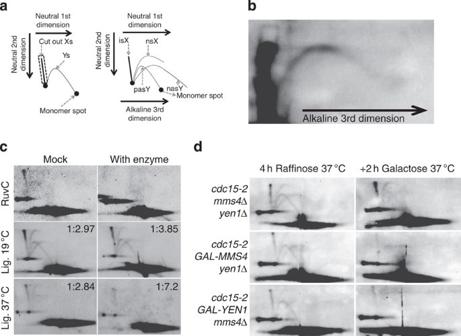Figure 5: The X-shaped DNA found in themms4Δyen1Δ telophase-blocked cells comprises the Holliday molecule with a discontinuity at the junction. (a) Schematic of the two strategies used to analyse by alkaline electrophoresis the physical nature of the NN-2D X-shaped spike. On the left, run a NN-2D and then run an alkaline electrophoresis for just the spike cut out of the gel. On the right, turn the NN-2D gel 90° and run a third alkaline dimension (NNA-3D). The expected ssDNA species in the NNA-3D are depicted: isX, intact full-length strands coming from the Xs; nsX, strands of a smaller size due to a nick (or a small gap) in the Xs; pasY, parental strands in the Y-shaped molecules; nasY, nascent strands in the Y-shaped molecules. (b) Several parallel two NN-2D as the one shown inFig. 4bwere run for themms4Δyen1Δ double mutant in 0.004% (v/v) MMS and, using the Southern blot of one of them as a reference, the expected location of the X-shaped molecule was cut out of the second gel and run under alkali conditions to analyse the four strands in the Xs (see also text andSupplementary Fig. 7). A representative result is shown. (c) NNA-3Ds for the telophase-blockedmms4Δyen1Δ double mutant afterin vitrotreatment of the agarose embedded DNA with the DNA processing enzymes RuvC and T4 DNA ligase. Mock denotes parallel treatments in which the enzymes were omitted. The nsX versus isX ratio of the ligase treatments is indicated at the upper-right corner of the corresponding pictures. (d) NNA-3Ds for an endonuclease induction experiment as the one shown inFig. 4c. Figure 5: The X-shaped DNA found in the mms4 Δ yen1 Δ telophase-blocked cells comprises the Holliday molecule with a discontinuity at the junction. ( a ) Schematic of the two strategies used to analyse by alkaline electrophoresis the physical nature of the NN-2D X-shaped spike. On the left, run a NN-2D and then run an alkaline electrophoresis for just the spike cut out of the gel. On the right, turn the NN-2D gel 90° and run a third alkaline dimension (NNA-3D). The expected ssDNA species in the NNA-3D are depicted: isX, intact full-length strands coming from the Xs; nsX, strands of a smaller size due to a nick (or a small gap) in the Xs; pasY, parental strands in the Y-shaped molecules; nasY, nascent strands in the Y-shaped molecules. ( b ) Several parallel two NN-2D as the one shown in Fig. 4b were run for the mms4 Δ yen1 Δ double mutant in 0.004% (v/v) MMS and, using the Southern blot of one of them as a reference, the expected location of the X-shaped molecule was cut out of the second gel and run under alkali conditions to analyse the four strands in the Xs (see also text and Supplementary Fig. 7 ). A representative result is shown. ( c ) NNA-3Ds for the telophase-blocked mms4 Δ yen1 Δ double mutant after in vitro treatment of the agarose embedded DNA with the DNA processing enzymes RuvC and T4 DNA ligase. Mock denotes parallel treatments in which the enzymes were omitted. The nsX versus isX ratio of the ligase treatments is indicated at the upper-right corner of the corresponding pictures. ( d ) NNA-3Ds for an endonuclease induction experiment as the one shown in Fig. 4c . Full size image The persistence of linkages between sister chromatids in anaphase is broadly believed to lead to a catastrophic mitosis. Previously, many reports using the model organism S. cerevisiae have shown that anaphase bridges form when these linkages comprise topological catenations, unresolved cohesion or unfinished replication [1] , [2] , [3] , [4] , [5] . Now, we show that this phenotype can be extended to the persistence of unresolved recombination intermediates (inter-sister JMs). We critically demonstrate this by controlling the activity of two of the SSEs that deal with these JMs (Mus81-Mms4 and Yen1) and then measuring chromosome segregation at the distal regions of the chromosome arm that carries the hot-spot locus for spontaneous JMs (the rDNA locus at cXIIr) ( Figs 1 , 2 , 3 , 4 , 5 ). Importantly, we provide several additional evidences that support the statement that unresolved inter-sister JMs cause anaphase bridges. First, the cXIIr missegregation observed in the absence of both Mus81-Mms4 and Yen1 depends on a functional HR pathway. Second, the cXIIr missegregation is reverted upon activation of either SSE in telophase. Third, increasing the steady–state levels of JMs by low doses of MMS boosts the presence of anaphase bridges (for example, visible by DAPI staining), which can nevertheless be still reverted in telophase by either SSE. Fourth, we directly visualize the presence of JMs at the rDNA and correlate their levels with the observed degree of cXIIr missegregation (both in the absence of the SSEs and after their reactivation in telophase). It is worth mentioning that it was not until very recently that several reports have been able to visualize DAPI-stained anaphase bridges when knocking down several SSEs in human-derived cell lines [30] , [31] . However, it was not clear whether these bridges linked sister chromatids and whether they actually comprise JMs or, else, they might be formed by unreplicated DNA as it has been suggested in MUS81-EME1-related ultra-fine anaphase bridges [55] . A surprising finding in our study was the negligible genetic interactions that Slx4 showed with the other two SSEs. In higher eukaryotes, SLX4 has been proposed as a central scaffold protein where different branched DNA-processing activities can be assembled, including JM-resolving activities by MUS81-EME1 and SLX1 (refs 30 , 31 , 32 , 33 ). At first, we believed this might reflect a difference between higher eukaryotes and yeast in accordance with reports showing a lack of interactions between Slx4 and Mus81-Mms4 (ref. 46 ). Nevertheless, another very recent report in this fast-moving field has pointed out that there is indeed an interaction bridged by Dpb11 (ref. 56 ). This raises new questions and suggests there may be two Mus81-Mms4 activities, being the Slx4-independent activity responsible for dealing with the JMs that led to SCBs in our hands. In contrast to Slx4, the clear genetic compensation between Mus81-Mms4 and Yen1 prompted us to deeply address the physical nature of the JMs that form the anaphase bridges. Strikingly, this study has uncovered some new and unexpected findings with important implication on the models of how HR bypasses SRFs. At present, there is a general consensus in that SRF-derived JMs are channelled towards iHJs that are then processed in pairs through the double HJ (dHJ) dissolution pathway, a job carried out by the Sgs1-Top3-Rmi1 (STR) helicase–topoisomerase complex [12] . However, there is also evidence that not all JMs can be resolved by STR. Recently, it has been hypothesized that the prominent mitotic STR-refractory JM is the nHJ [10] , [11] , which would be resolved by Mus81-Mms4 in G2/M [24] , [57] , [58] , [59] . The actual role of Yen1 is still controversial, although it has been recently shown to act after Mus81-Mms4 on those HJs that persist until anaphase (for example, single iHJs) [9] , [10] , [11] , [21] , [58] , [60] , [61] . Our in vivo results strongly support the nHJ hypothesis and the reported activity for Mus81-Mms4. Indeed, what we saw in telophase in the absence of both Mus81-Mms4 and Yen1 were noncanonical HJs carrying a discontinuity in one strand (either nHJs or HJs with small gaps, but clearly not iHJs). Surprisingly, these noncanonical HJ in an mms4 Δ background were almost fully resolved after Yen1 expression in anaphase ( Figs 4c and 5d ). The simplest explanation of these results in the context of the nHJs hypothesis would be that Mus81-Mms4 and Yen1 are both nHJ-resolvases ( Fig. 6 ). In agreement with this hypothesis, the in vitro specificity of Yen1 homologues in flies and humans is not restricted to iHJs [62] , [63] . Also, a very recent report using full-length yeast Yen1 supports at last significant in vitro activities against branched DNA structures other than iHJs, including nHJs [60] . An alternative possibility that would fit with Yen1 being just an iHJ-resolvase is that, in the absence of Mus81-Mms4, nHJs (and other discontinuous HJs) could be converted into iHJs and then process by Yen1 ( Fig. 6 ). This step would take place by either branch migration out of the nick or the action of a ligase/polymerase, and could be either biologically induced or being part of a dynamic equilibrium where the discontinuous HJ forms would act as metastable states. In favour of this latter scenario is the fact that Yen1 gets activated in anaphase and that Mus81-Mms4 specificity may also change at this cell cycle stage to resolve iHJs as well as nHJs [58] , [60] , [61] . Finally, we cannot completely rule out the possibility that these noncanonical HJs are formed in vitro during DNA extraction by branch migration towards a pre-existing nick, despite using controlled conditions known to minimize such migration [64] . Nevertheless, and in support of these non-canonical HJs being present in vivo , it is also worth mentioning a very recent report where HJs comprising clear gaps of ssDNA close to the junction were visualized by electron microscopy on an artificial chromosome in yeast [65] . 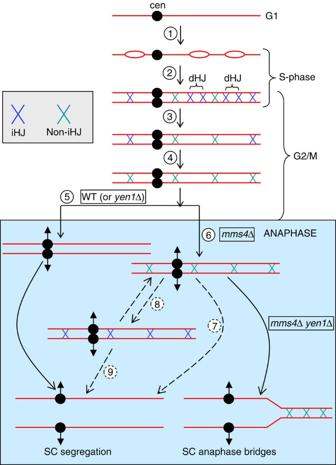Figure 6: Models of how Mus81-Mms4 and Yen1 might cooperate in anaphase to resolve anaphase bridges formed by nicked (and other discontinuous) Holliday junctions. Initially, stalled RFs in the previous S-phase are bypassed through the HR pathway, leaving behind JMs (steps 1 and 2). Some JMs can then be resolved by helicases through SDSA, whereas others end up as either iHJs or nHJs9,10,11. The Sgs1-dependent dHJ disolution pathway will then deal with much of the iHJs (step 3). Persistent nHJs, and probably other noncanonical HJs, would be processed by SSEs9,10,11. Persistent iHJs are in theory possible as well (for example, single iHJs). However, they must be eventually converted into nHJs (step 4) (Fig. 5). Mus81-Mms4 is normally sufficient to resolve all nHJs in G2/M (step 5), and only under replicative stress would Mus81-Mms4 become saturated (Fig. 1a). Two main models are possible to unlink the sister chromatids by Yen1 in the absence of Mus81-Mms4 or when it becomes saturated. If Yen1 resolves nHJsin vivoit would directly compensate for the Mus81-Mms4 deficiency (dashed lines, step 7). If Yen1 is just an iHJ resolvase (step 9), nHJ and other non-iHJ species necessarily need to be converted into iHJs at some point, for example, by branch migration, nick ligation, gap filling and so on (step 8). Figure 6: Models of how Mus81-Mms4 and Yen1 might cooperate in anaphase to resolve anaphase bridges formed by nicked (and other discontinuous) Holliday junctions. Initially, stalled RFs in the previous S-phase are bypassed through the HR pathway, leaving behind JMs (steps 1 and 2). Some JMs can then be resolved by helicases through SDSA, whereas others end up as either iHJs or nHJs [9] , [10] , [11] . The Sgs1-dependent dHJ disolution pathway will then deal with much of the iHJs (step 3). Persistent nHJs, and probably other noncanonical HJs, would be processed by SSEs [9] , [10] , [11] . Persistent iHJs are in theory possible as well (for example, single iHJs). However, they must be eventually converted into nHJs (step 4) ( Fig. 5 ). Mus81-Mms4 is normally sufficient to resolve all nHJs in G2/M (step 5), and only under replicative stress would Mus81-Mms4 become saturated ( Fig. 1a ). Two main models are possible to unlink the sister chromatids by Yen1 in the absence of Mus81-Mms4 or when it becomes saturated. If Yen1 resolves nHJs in vivo it would directly compensate for the Mus81-Mms4 deficiency (dashed lines, step 7). If Yen1 is just an iHJ resolvase (step 9), nHJ and other non-iHJ species necessarily need to be converted into iHJs at some point, for example, by branch migration, nick ligation, gap filling and so on (step 8). Full size image In conclusion, the structure-selective nucleases Mus81-Mms4 and Yen1, but not Slx1-Slx4, play an overlapping role in preventing and resolving a novel type of stable sister chromatid anaphase bridges formed by noncanonical and discontinuous forms of the Holliday junction molecule. In addition, we show that these unresolved recombination intermediates do not break apart when cells reach anaphase in the absence of both Mus81-Mms4 and Yen1. This sheds new light on the physical nature of anaphase bridges and the HJ molecule in eukaryotes as well as the physiological roles of the eukaryotic structure-selective nucleases. Yeast strains and experimental conditions All yeast strains used in this work are listed in Supplementary Table 1 . Parental S288C strain carrying the cdc15-2 allele, the tetOs array at cXIIr-Tel ( tetOs:1061 ) and the TetR-YFP fusion has been described elsewhere [36] . Gene deletions, marker swaps and allele/promoter replacements were engineered using PCR methods. All strains were grown overnight in air orbital incubators at 25 °C in YEPD media unless stated otherwise. G1-to-telophase experiments were performed as follows: asynchronous cultures were first adjusted to OD 600 =0.5, then synchronized in G1 at 25 °C for 3 h by adding 50 ng ml −1 of alpha-factor (all tested strains were bar1 Δ), and finally released from the G1 arrest at 37 °C for 4 h. For the G1 release, cells were washed twice and resuspended in fresh media containing 0.1 mg ml −1 of pronase E. When indicated, DNA damage was induced at the time of the G1 release by adding MMS. MMS was kept in the media until the telophase arrest and removed in such instances where cells were released from telophase to measure viability. In the dose–response experiments, cell cultures were split into ten flasks at the time of the G1 release and nine 1:3 serial dilutions of MMS were used. The MMS final concentrations ranged from 0.1 to 0.000015% (v/v). The tenth culture was left without MMS as a control. When galactose induction of the SSE genes was required, cells were grown in YP raffinose 2% (w/v). Raffinose was also used as the carbon source all through the G1-to-telophase synchronous cell cycle, and galactose was added at 2% (w/v) at the time of the cdc15-2 telophase block while keeping the yeast culture at 37 °C. Cell viability was measured by plotting number of colonies grown on YPD plates after 3 days at 25 °C relative to total cell number counted by a haemocytometer at the time of platting. Error bars in all graphs represent the s.e.m. of independent technical replicates. The number of replicates ( N ) is indicated either in the figure legends or in the main text. Single-cell analyses by flow cytometry and microscopy Flow cytometry to follow up bulk DNA replication was carried out taking 300 μl of culture in 0.9 ml 100% ethanol. Cells were pelleted and resuspended in 1 × SSC buffer with 0.01 mg ml −1 of RNaseA and incubated overnight at 37 °C. Fifty microlitres of 1 × SSC with 1.2 mg ml −1 of proteinase K was added and incubated at 50 °C for 1 h. After that, 500 μl of 1 × SSC with propidium iodine 3 μg ml −1 was added and incubated at room temperature for 1 h. Samples were analysed using a BD FACScalibur machine [36] . Cell cycle progression and cXIIr segregation were analysed by wide-field fluorescence microscopy [36] . A stack of 20 z-focal plane images (0.3 μm depth) was collected on a Leica DMI6000, using a 63 × /1.30 immersion objective and an ultrasensitive DFC 350 digital camera, and processed with the AF6000 software (Leica). Gross DNA masses were stained for microscopy using DAPI at 1 μg ml −1 final concentration in a 0.25% (v/v) Triton X-100 solution. The staining was performed right before visualization under the microscope in cell pellets previously frozen at −20 °C for 48 h. Analyses of branched DNA structures and chromosome integrity PFGE was used as the standard procedure to determine the presence of branched DNA structures at the chromosome level and also to quantify the changes among different strains, treatments and/or chromosomes [21] , [48] . Two-dimensional neutral-neutral (NN-2D) and three-dimensional neutral-neutral-alkaline (NNA-3D) DNA electrophoresis were, respectively, used to study whether branched DNA corresponded to the HJ molecule and to distinguish between intact and discontinuous HJs [52] . Yeast DNA for PFGE, NN-2D and NNA-3D was prepared in low-melting agarose plugs in conditions known to avert branch migration and preserve non-linear forms with no need of using psoralen to crosslink [64] . In brief, 4 ml of OD 600 =1 was pelleted and embedded into a 0.5% (w/v) agarose plug. Chromosome-sized DNA was obtained after subsequent overnight digestions of the plug with lyticase (2,500 units ml −1 ), RNaseA (0.5 units ml −1 ) and Proteinase K (1 mg ml −1 ). All digestions were carried out at 37 °C (including the Proteinase K step) to minimize the heat-labile in vitro DNA shearing reported for MMS and any remaining migration of the branched DNA structures [43] , [64] . PFGE to see yeast chromosomes was performed using a CHEF DR-III system (Bio-Rad) in a 0.8% (w/v) agarose gel made with 0.5 × TBE buffer and run at 12 °C for 20 h at 6 V cm −1 with an initial switching time of 80 s, a final of 150 s and an angle of 120°. PFGE to resolve better the chromosome XII ( Fig. 3b ) was performed at 3 V cm −1 for 68 h with 300 and 900 s of initial and final switching time, respectively [36] . Yeast chromosomes were visualized after staining with ethidium bromide and quantified with the QuantityOne software (Bio-Rad). To specifically visualize the chromosome XII, a Southern blot was carried out by a saline downwards transference onto positively charged membranes (Roche), followed by hybridization with a fluorescein-labelled probe (Roche) that covers both ITS regions within the rDNA unit. Detection was performed by chemiluminescence using an anti-fluorescein antibody coupled to alkaline phosphatase (Roche) and using CDP-star (Roche) as the substrate. DNA NN-2D and NNA-3D electrophoresis to visualize JMs were carried out as following. First, the agarose plug was treated with the Proteinase K inhibitor Pefablock (Roche) at 1 mg ml −1 followed by overnight digestion with 1,500 units ml −1 of the restriction enzyme BglII (New England Biolabs). Then, one-half of the plug was loaded onto a 0.35% (w/v) agarose gel and the first dimension run at 0.8 V cm −1 for 24 h. Next, the corresponding lane was sliced, re-oriented 90° anticlockwise and the second dimension was run in a 1% (w/v) agarose gel at 6 V cm −1 for 9 h under the presence of 0.3 μg ml −1 of ethidium bromide in both the gel and the running buffer. Importantly, the buffer was left recirculating through a cooling system to keep constant the running temperature at 16 °C. For NN-2D, the gel was then transferred to a positively charged membrane (Roche) for Southern blot analysis. In the case of NNA-3D [52] , the agarose gel obtained after the NN-2D procedure was first soaked in 0.04 N NaOH plus 2 mM EDTA five times for 1 h each for alkaline equilibration. Then, a third electrophoresis was run in the same orientation as the first one was. The running conditions for this ‘third dimension’ were 0.8 V cm −1 for 38 h at 16 °C. Then, this 3D gel was used for Southern blot analysis. Before transference onto the membrane, a neutralization step was added before depurination just for this gel. The same procedure was followed when the X-shaped structure was cut out right after the NN-2D. In the case of treatment with RuvC (Abcam) we followed a procedure similar to a previous report [66] . Thus, we first washed the agarose plug in RuvC buffer for 30 min at room temperature and then washed once for 30 min at 4 °C. Then the plugs were incubated in 150 μl of buffer with 3 μg RuvC for 4 h at 4 °C and then 1 h at 55 °C. In the case of treatment with T4 DNA ligase, we employed an adaptation of the RuvC protocol for this enzyme, taking also into account general protocols for the T4 ligase. Thus, we washed in T4 ligase buffer for 30 min at room temperature and then washed once in T4 ligase buffer for 30 min at 4 °C. Then the plugs were incubated in 150 μl of buffer with 3,500 cohesive end units of T4 DNA ligase either at 19 °C or 37 °C. The same procedures but without enzymes (mock) were followed with another plug as negative controls. Southern blots of NN-2D and NNA-3D were carried out by a saline upwards transference followed by hybridization with the same fluorescein-labelled probe we used for PFGE. For quantifications of the X-shaped DNA molecules in the NN-2D, we took photos of the emitted light in a ChemiDoc MP apparatus (BioRad) and used the software ImageLab (BioRad). We picked a time exposure in all cases (360 s) where the signal of the X-shaped molecules was visible but not saturated. We then picked another time exposure for all linear 1N DNA signals where they were not saturated either (1 s). The 1N signals include the monomer spot and the smear that appeared during the first dimension (this smear is due to overloading and is frequently stronger from samples embedded in agarose plugs). In 28% of our NN-2Ds, the 1N signal also included a second smear trailing from the monomer spot in the second dimension, which has been previously defined as an artefact [67] . Finally, we calculated the quotient [background−subtracted intensity of the Xs/background−subtracted intensity of the 1N] and established the 100% signal as the one in the telophase-blocked cdc15-2 mms4 Δ yen1 Δ strain in raffinose. To calculate the relative amount of discontinuous HJs over the whole of X-shaped molecules, we directly quantified the ssDNAs resolved from the X-shaped structure after the NNA-3Ds according to the following formulae: [background−subtracted intensity of the full-length ssDNA line/background−subtracted intensity of the arc for smaller ssDNAs]. A ratio of 3:1 would be expected if all X-shaped structures were discontinuous HJs ( Supplementary Fig. 7 ). How to cite this article: García-Luis, J. and Machín, F. Mus81-Mms4 and Yen1 resolve a novel anaphase bridge formed by noncanonical Holliday junctions. Nat. Commun. 5:5652 doi: 10.1038/ncomms6652 (2014).